A20 controls intestinal homeostasis through cell-specific activities The transcription factor NF-κB is indispensable for intestinal immune homeostasis, but contributes to chronic inflammation and inflammatory bowel disease (IBD). A20, an inhibitor of both NF-κB and apoptotic signalling, was identified as a susceptibility gene for multiple inflammatory diseases, including IBD. Despite absence of spontaneous intestinal inflammation in intestinal epithelial cell (IEC) specific A20 knockout mice, we found additional myeloid-specific A20 deletion to synergistically drive intestinal pathology through cell-specific mechanisms. A20 ensures intestinal barrier stability by preventing cytokine-induced IEC apoptosis, while A20 prevents excessive cytokine production in myeloid cells. Combining IEC and myeloid A20 deletion induces ileitis and severe colitis, characterized by IEC apoptosis, Paneth and goblet cell loss, epithelial hyperproliferation and intestinal microbiota dysbiosis. Continuous epithelial cell death and regeneration in an inflammatory environment sensitizes cells for neoplastic transformation and the development of colorectal tumours in aged mice. Inflammatory bowel disease (IBD) is a chronic inflammatory disorder of the gastrointestinal tract and includes Crohn’s disease (CD) and ulcerative colitis (UC) as the main phenotypes. The aetiology of IBD is complex and involves interactions between genetic factors, environmental triggers including the intestinal microbiota and the host immune system. It is generally acknowledged that IBD arises as a result of the loss of tolerance towards the normal intestinal microbiota due to a hyperactive immune response and/or an instable mucosal barrier [1] . One of the consequences of chronic intestinal inflammation is the promotion of tumorigenesis, and patients with IBD have a higher risk of developing colitis-associated cancer (CAC) [2] . Genome-wide association studies and immunochip analysis have up to now identified 163 IBD-associated loci, many of them involved in immune regulation and epithelial barrier function, including the NF-κB inhibitory protein A20 (also known as TNFAIP3) [3] , [4] , [5] , [6] . The transcription factor NF-κB has crucial roles in intestinal homeostasis and pathology. On one hand, NF-κB contributes to IBD development as a mediator of pro-inflammatory responses, predominantly in the myeloid cells. On the other hand, NF-κB activity in epithelial cells has a protective role through the expression of anti-apoptotic proteins, antimicrobial peptides and mucus, thus enhancing the epithelial barrier function [7] . An important protective factor in the intestinal epithelium is the NF-κB-inducible protein A20. Mice with enterocyte-specific A20 deletion (A20 IEC-KO ) are hypersensitive to dextran sodium sulphate-induced colitis and to tumour necrosis factor (TNF)-induced epithelial apoptosis and lethality [8] . Although A20 is indispensable to maintain barrier integrity in conditions of inflammation, A20 IEC-KO mice do not spontaneously develop intestinal inflammation [8] . Similarly, although mice with myeloid cell-specific deletion of A20 (A20 myel-KO ) develop rheumatoid arthritis-like symptoms due to excessive NF-κB activation and inflammatory responses, they do not develop spontaneous intestinal pathology [9] . The absence of any spontaneously developing intestinal phenotype in A20 IEC-KO or A20 myel-KO may therefore question the role of A20 in human IBD as originally suggested by human genetic studies [4] , [5] , [6] . However, we here show that spontaneous intestinal pathology develops when mice are deficient for A20 in both intestinal epithelial cells (IECs) and myeloid cells. A20 IEC/myel-KO mice not only produce high levels of inflammatory cytokines, but also develop spontaneous intestinal inflammation characterized by increased epithelial apoptosis and hyperproliferation. A20 IEC/myel-KO mice progressively lose their Paneth and goblet cells leading to defective antimicrobial peptide and mucus production, bacterial infiltration and severe colitis in aged mice. Over time, A20 IEC/myel-KO mice develop hyperplastic and dysplastic epithelium which displays typical hallmarks of human colorectal cancer, including hyperactive Wnt signalling and aberrant stem cell marker expression. A20 IEC/myel-KO mice develop spontaneous intestinal defects We have previously shown that A20 IEC-KO mice do not show any spontaneous phenotype but are hypersensitive to experimental colitis associated with increased IEC apoptosis [8] . In contrast, A20 myel-KO mice develop rheumatoid arthritis-like symptoms, but not colitis, due to hyperactivated myeloid cells producing elevated levels of inflammatory cytokines, including TNF and interleukin-6 (IL-6) (ref. 9 ). Combined IEC and myeloid A20 deficiency (A20 IEC/myel-KO ) fully recapitulates the inflammatory phenotype of A20 myel-KO mice, showing myeloid cell expansion with lymphadenopathy and splenomegaly, and increased levels of TNF and IL-6 in their serum ( Supplementary Fig. 1 ). In contrast to wild-type control, A20 myel-KO and A20 IEC-KO mice, A20 IEC/myel-KO mice spontaneously develop colitis symptoms, as revealed by histological and stool colitis scoring ( Fig. 1a ). Intestinal inflammation is rather mild in young A20 IEC/myel-KO mice but progresses to ileitis and moderately active chronic colitis in aged mice ( Supplementary Fig. 2 ). Histological analysis of distal ileal segments showed severe depletion of granular Paneth cells in crypts of A20 IEC/myel-KO mice in contrast to crypts of wild-type mice, as revealed by Alcian-blue-PAS (AB-PAS) staining ( Fig. 1b ) or immunostaining for lysozyme ( Fig. 1c ). In addition, in situ hybridization of Paneth cell-specific cryptidine-1 (Crypt-1) on ileal sections shows strong and homogeneous Crypt-1 expression in wild-type mice, while Crypt-1 expression is compromised in crypts of A20 IEC/myel-KO mice ( Fig. 1d ). Expression analysis of Paneth cell-specific Crypt-1 and lysozyme-P (LysP) by quantitative PCR on ileal epithelial cell lysates shows dramatically reduced expression levels in A20 IEC/myel-KO mice compared with wild-type controls ( Fig. 1e ). Next to Paneth cell defects, A20 IEC/myel-KO mice also display substantially reduced numbers of mucus-producing goblet cells. Carnoy fixed colon samples from wild-type, A20 IEC-KO , A20 myel-KO and A20 IEC/myel-KO mice were used for Muc-2 immunostaining and bacterial 16S FISH [10] to visualize the bacterial epithelial interface. Intestinal bacteria are separated from the epithelium by a sterile mucous layer of approximately 40 μm thick in wild-type, A20 IEC-KO and A20 myel-KO mice, whereas in A20 IEC/myel-KO mice the mucous layer is significantly thinner and often interrupted, allowing closer interaction between bacteria and epithelial cells ( Fig. 1f,g ). In agreement, the expression of goblet cell-specific Muc-2 expression is significantly reduced, as shown by quantitative PCR on colon samples from A20 IEC/myel-KO mice ( Fig. 1h ). Together, these data demonstrate the spontaneous development of intestinal inflammation and epithelial defects, including early loss of Paneth and goblet cells in A20 IEC/myel-KO mice. 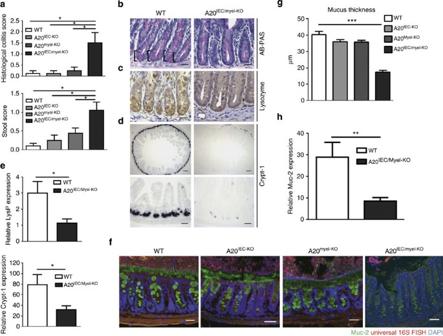Figure 1: A20IEC/myel-KOmice develop spontaneous intestinal defects. (a) Clinical colitis scores on the basis of histological (hist., upper graph) and stool (lower graph) colitis parameters of naive 10–30-week-old A20IEC-KO(hist. scoren=8, stool scoren=12), A20myel-KOmice (hist. scoren=8, stool scoren=16), A20IEC/myel-KOmice (hist. scoren=8, stool scoren=18) and control wild-type (WT) littermate mice (hist. scoren=8, stool scoren=15). All A20IEC/myel-KOmice display colitis histopathology and mild stool colitis scores. (b) AB-PAS staining of ileal sections from 30-week-old A20IEC/myel-KOand wild-type (WT) control littermates. The crypt base region with highly granular Paneth cells in WT section is indicated by square brackets (Scale bars, 20 μm). (c) Immunostaining of ileal sections using an antibody-recognizing lysozyme in intracellular granules of Paneth cells (Scale bars, 20 μm). (d)In situhybridization on ileal sections using a specific probe recognizing Crypt-1 transcripts (Scale bars, upper: 150μm, lower: 50 μm). (e) Quantitative PCR analysis for LysP and Crypt-1 on IEC lysates from the small intestine from 12-week-old wild-type (WT,n=5) and A20IEC/myel-KO(n=9) mice. (f) Immunofluorescent staining for Muc-2 and 16S bacterial FISH on colon sections from 20-week-old A20IEC-KO, A20myel-KOmice, A20IEC/myel-KOand control wild-type (WT) littermate mice (Scale bars, 50 μm). (g) Thickness of bacterium-free mucus layer of colon tissue of wild-type (WT,n=9), A20IEC-KO(n=8), A20myel-KO(n=10) and A20IEC/myel-KOmice (n=9). (h) Quantitative PCR analysis for Muc-2 on IEC colon lysates from 30-week-old wild-type (WT,n=5) and A20IEC/myel-KO(n=8) mice. Error bars represent s.e.m. *P<0.05, **P<0.01, ***P<0.001 using Student’st-test. Figure 1: A20 IEC/myel-KO mice develop spontaneous intestinal defects. ( a ) Clinical colitis scores on the basis of histological (hist., upper graph) and stool (lower graph) colitis parameters of naive 10–30-week-old A20 IEC-KO (hist. score n =8, stool score n =12), A20 myel-KO mice (hist. score n =8, stool score n =16), A20 IEC/myel-KO mice (hist. score n =8, stool score n =18) and control wild-type (WT) littermate mice (hist. score n =8, stool score n =15). All A20 IEC/myel-KO mice display colitis histopathology and mild stool colitis scores. ( b ) AB-PAS staining of ileal sections from 30-week-old A20 IEC/myel-KO and wild-type (WT) control littermates. The crypt base region with highly granular Paneth cells in WT section is indicated by square brackets (Scale bars, 20 μm). ( c ) Immunostaining of ileal sections using an antibody-recognizing lysozyme in intracellular granules of Paneth cells (Scale bars, 20 μm). ( d ) In situ hybridization on ileal sections using a specific probe recognizing Crypt-1 transcripts (Scale bars, upper: 150μm, lower: 50 μm). ( e ) Quantitative PCR analysis for LysP and Crypt-1 on IEC lysates from the small intestine from 12-week-old wild-type (WT, n =5) and A20 IEC/myel-KO ( n =9) mice. ( f ) Immunofluorescent staining for Muc-2 and 16S bacterial FISH on colon sections from 20-week-old A20 IEC-KO , A20 myel-KO mice, A20 IEC/myel-KO and control wild-type (WT) littermate mice (Scale bars, 50 μm). ( g ) Thickness of bacterium-free mucus layer of colon tissue of wild-type (WT, n =9), A20 IEC-KO ( n =8), A20 myel-KO ( n =10) and A20 IEC/myel-KO mice ( n =9). ( h ) Quantitative PCR analysis for Muc-2 on IEC colon lysates from 30-week-old wild-type (WT, n =5) and A20 IEC/myel-KO ( n =8) mice. Error bars represent s.e.m. * P <0.05, ** P <0.01, *** P <0.001 using Student’s t -test. Full size image IEC apoptosis and hyperproliferation in A20 IEC/myel-KO mice Tissue analysis by transmission electron microscopy of ileal crypts from wild-type mice shows Paneth cells containing large intracellular vacuoles alternated by intestinal stem cells ( Fig. 2a ). Ileal crypts of A20 IEC/myel-KO mice, however, are devoid of granular Paneth cells, and individual stem cells cannot be identified on the basis of morphology only ( Fig. 2a ). In addition, crypt regions of A20 IEC/myel-KO mice contain phagocytosed dead cell fragments, which stain positive for TUNEL and cleaved caspase-3 indicating that A20 IEC/myel-KO crypt cells undergo apoptosis ( Fig. 2b,c ). Quantification of active caspase-3 positive cells reveals significantly increased numbers of apoptotic cells in both ileum and colon of A20 IEC/myel-KO mice ( Fig. 2d ). Next, epithelial cell proliferation was determined by Ki67 immunohistochemistry. Slow cycling stem cells, which are only sporadically Ki67 + , are positioned at the crypt bottom and give rise to active cycling (high Ki67 + ) transit amplifying cells which are located above the stem cell/Paneth cell compartment in the small intestine of wild-type mice ( Fig. 2e ) [11] . In A20 IEC/myel-KO mice, however, proliferating (Ki67 + ) active cycling cells occupy the entire crypts including the crypt bottoms ( Fig. 2e ). Since Paneth cells support intestinal stem cells by producing trophic factors [12] , we wondered if Paneth cell loss had a direct impact on the stem cell compartment. In situ hybridization for the small intestinal stem cell marker olfactomedin-4 (Olfm4) shows comparable Olfm4 expression in the crypts of A20 IEC/myel-KO mice compared with crypts from wild-type mice ( Fig. 2f ), indicating that the stem cell compartment is not affected in A20 IEC/myel-KO mice. In addition, changes in expression of intestinal stem cell markers could not be observed in the small intestine of A20 IEC/myel-KO mice compared with wild-type mice ( Supplementary Fig. 3 ). Together, these data show that Paneth cell deficiency does not affect normal stem cell numbers and suggest redundant mechanisms for stem cell support in the small intestine of A20 IEC/myel-KO mice. Similar to our observations in the small intestine, increased apoptosis in the colon ( Fig. 2b–d ) is accompanied by increased cell proliferation as shown by Ki67 immunohistochemistry ( Fig. 2e ). While cell proliferation is confined to the colonic crypt bottom in wild-type mice, proliferating cells in A20 IEC/myel-KO mice populate almost the entire elongated crypts ( Fig. 2e ). In conclusion, A20 IEC/myel-KO mice display increased IEC apoptosis and proliferation in both the small and large intestine. 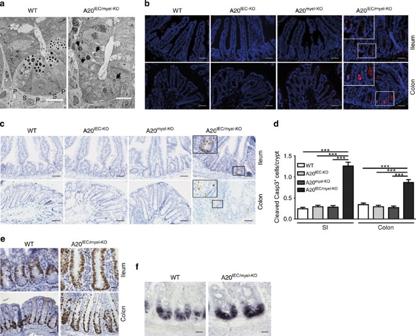Figure 2: IEC apoptosis and hyperproliferation in A20IEC/myel-KOmice. (a) Transmission electron micrographs of small intestinal crypt region of wild-type (WT) and A20IEC/myel-KOmice. Arrows indicate condensed phagocytosed dead cell remnants (Scale bars, 4 μm) (S=stem cell, P=Paneth cell). (b,c) Representative TUNEL staining (b) and immunostaining of active caspase-3 (c) in crypts of the terminal ileum and colon of wild-type (WT), A20IEC-KO, A20myel-KOand A20IEC/myel-KOmice (Scale bars, 50 μm). (d) Quantification of cleaved caspase-3 positive cells in crypts of wild-type (WT,n=5), A20IEC-KO(n=5), A20myel-KO(n=5) and A20IEC/myel-KOmice (n=5). Error bars represent s.e.m. ***P<0.001 using Student’st-test. (e) Ki67 immunostaining on wild-type (WT) and A20IEC/myel-KOileal crypts (Scale bars, 5 μm). (f)In situhybridization for Olfm4 on wild-type (WT) and A20IEC/myel-KOileal crypts using an Olfm4 specific probe (Scale bars, 5 μm). Figure 2: IEC apoptosis and hyperproliferation in A20 IEC/myel-KO mice. ( a ) Transmission electron micrographs of small intestinal crypt region of wild-type (WT) and A20 IEC/myel-KO mice. Arrows indicate condensed phagocytosed dead cell remnants (Scale bars, 4 μm) (S=stem cell, P=Paneth cell). ( b , c ) Representative TUNEL staining ( b ) and immunostaining of active caspase-3 ( c ) in crypts of the terminal ileum and colon of wild-type (WT), A20 IEC-KO , A20 myel-KO and A20 IEC/myel-KO mice (Scale bars, 50 μm). ( d ) Quantification of cleaved caspase-3 positive cells in crypts of wild-type (WT, n =5), A20 IEC-KO ( n =5), A20 myel-KO ( n =5) and A20 IEC/myel-KO mice ( n= 5). Error bars represent s.e.m. *** P <0.001 using Student’s t -test. ( e ) Ki67 immunostaining on wild-type (WT) and A20 IEC/myel-KO ileal crypts (Scale bars, 5 μm). ( f ) In situ hybridization for Olfm4 on wild-type (WT) and A20 IEC/myel-KO ileal crypts using an Olfm4 specific probe (Scale bars, 5 μm). Full size image A20-deficient Paneth cells undergo cytokine-induced apoptosis Wnt signalling is essential for Paneth cell maturation [13] , [14] , [15] suggesting that disturbed Wnt signalling might contribute to reduced Paneth cell numbers in A20 IEC/myel-KO mice. Although A20 has recently been suggested to restrict Wnt signalling in the intestinal epithelium by binding to the β-catenin destruction complex supporting β-catenin ubiquitination and degradation [16] , normal β-catenin and Sox9 expression is observed on sections from small intestinal tissue from A20 IEC/myel-KO mice ( Supplementary Fig. 4a,b ). In addition, wild-type and A20-deficient organoids stimulated with Wnt3a for 6 h show similar expression of Wnt target genes Cyclin-D1 and c-Myc ( Supplementary Fig. 4c ). Together these data indicate that A20 deficiency does not affect Wnt signalling and gene expression in vitro and in vivo . To assess whether A20 IEC/myel-KO mice have inherent crypt defects or develop these defects progressively, ileal sections from A20 IEC/myel-KO mice of different age were analysed. In contrast to 5-week-old A20 IEC/myel-KO mice, which have mature Crypt-1 expressing Paneth cells in the intestinal crypts, the number of Paneth cells drastically drops around the age of 10 to 15 weeks ( Fig. 3a ). In contrast to the reduction in Crypt-1 expression, Olfm4 expression stays relatively stable in mice of different age ( Fig. 3b ), indicating that Paneth cell loss does not strongly affect intestinal stem cell populations. Immunohistochemical staining for the Paneth cell marker lysozyme in combination with TUNEL, identifying apoptotic cells, confirmed the impaired survival of Paneth cells in A20 IEC/myel-KO mice. While crypts of 5-week-old A20 IEC/myel-KO mice do not show signs of apoptosis, most crypts of older A20 IEC/myel-KO mice display apoptotic cells, often colocalizing with epithelial lysozyme, indicative of Paneth cells ( Fig. 3c ). Twenty-week-old A20 IEC/myel-KO mice have severely reduced Paneth cell numbers in their crypts ( Fig. 3c ). In agreement with the progressive loss of Paneth cells in A20 IEC/myel-KO mice, we observed an age-dependent reduction in antimicrobial LysP and Crypt-1 peptide expression in the ileal epithelial lysates ( Fig. 3d ). Interestingly, Paneth cell apoptosis coincides with the mucosal accumulation of lysozyme-positive myeloid cells ( Fig. 3c ), suggesting that cytokines released by recruited A20-deficient myeloid cells may induce Paneth cell apoptosis. In line with this, increasing amounts of the inflammatory cytokines IL-6 and TNF could be measured in serum from A20 IEC/myel-KO mice of different age ( Fig. 3e ). The hypersensitivity of A20-deficient Paneth cells to apoptosis could be confirmed in A20 IEC-KO mice exposed to TNF. Unchallenged A20 IEC-KO mice have a normal crypt architecture with normal Paneth cell numbers [8] . When injecting a sublethal dose of recombinant TNF, apoptosis of crypt cells including Paneth cells can be observed ( Supplementary Fig. 5a ). Twenty four hours after injection, Paneth cells are strongly reduced. In agreement, quantification of LysP and Crypt-1 expression by quantitative PCR shows strong reduction of both Paneth cell markers after TNF exposure ( Supplementary Fig. 5b ). Finally, in vitro studies on intestinal organoid cultures confirmed the above findings in mice. Stimulation of organoid cultures derived from wild-type and A20 IEC-KO mice with recombinant TNF or IFNγ, induces complete disintegration of A20-deficient organoids, in contrast to wild-type organoids which remain largely unaffected ( Fig. 3f , Supplementary Movies 1 and 2 ). Moreover, lysozyme immunostaining for Paneth cells combined with TUNEL or cleaved caspase-3, demonstrates Paneth cell apoptosis in A20-deficient organoid cultures exposed to TNF ( Fig. 3g and Supplementary Fig. 6 ). Similar observations were done on exposure of organoids to IFNγ ( Fig. 3g and Supplementary Fig. 6 ). In conclusion, Paneth cells in A20 IEC/myel-KO mice undergo progressive cell death induced by cytotoxic cytokines including TNF and IFNγ. 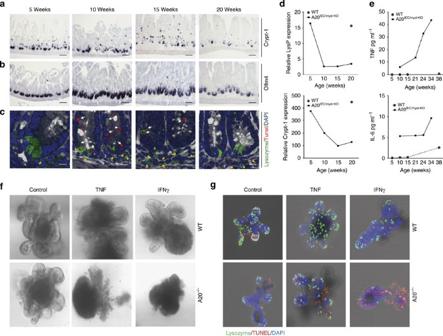Figure 3: A20-deficient Paneth cells are progressively lost by apoptosis. (a,b)In situhybridization on ileal sections of A20IEC/myel-KOmice using a specific probe recognizing Crypt-1 (a) and Olfm4 (b) transcripts (Scale bars, 50 μm). (c) Immunofluorescent staining for TUNEL (red) and Lysozyme (green) on ileal sections of A20IEC/myel-KOmice. White arrows: TUNEL-positive cells, Yellow arrows: Lysozyme-positive leukocytes (Scale bars, 5 μm). (d) Quantitative PCR analysis for Lysozyme-P (LysP) and Crypt-1 on ileal IEC lysates from wild-type (WT) and A20IEC/myel-KOmice of different age. (e) Levels of IL-6 and TNF in serum from wild-type (WT) and A20IEC/myel-KOmice of different age. (f) Representative pictures of wild-type (WT) and A20−/−intestinal organoids after 18 h stimulation with vehicle (control), TNF or IFNγ (10 ng ml−1). (g) Representative immunofluorescent pictures for detection of TUNEL (red) and Lysozyme (green) in wild-type (WT) and A20−/−gut organoids 4 h after stimulation with vehicle (control), TNF or IFNγ. Figure 3: A20-deficient Paneth cells are progressively lost by apoptosis. ( a , b ) In situ hybridization on ileal sections of A20 IEC/myel-KO mice using a specific probe recognizing Crypt-1 ( a ) and Olfm4 ( b ) transcripts (Scale bars, 50 μm). ( c ) Immunofluorescent staining for TUNEL (red) and Lysozyme (green) on ileal sections of A20 IEC/myel-KO mice. White arrows: TUNEL-positive cells, Yellow arrows: Lysozyme-positive leukocytes (Scale bars, 5 μm). ( d ) Quantitative PCR analysis for Lysozyme-P (LysP) and Crypt-1 on ileal IEC lysates from wild-type (WT) and A20 IEC/myel-KO mice of different age. ( e ) Levels of IL-6 and TNF in serum from wild-type (WT) and A20 IEC/myel-KO mice of different age. ( f ) Representative pictures of wild-type (WT) and A20 −/− intestinal organoids after 18 h stimulation with vehicle (control), TNF or IFNγ (10 ng ml −1 ). ( g ) Representative immunofluorescent pictures for detection of TUNEL (red) and Lysozyme (green) in wild-type (WT) and A20 −/− gut organoids 4 h after stimulation with vehicle (control), TNF or IFNγ. Full size image Severe colitis and colorectal tumour development in aged A20 IEC/myel-KO mice We have shown that A20 IEC/myel-KO mice have a compromised intestinal barrier due to epithelial apoptosis and progressive Paneth and goblet cell loss, which facilitates bacterial epithelial interaction and infiltration, likely further enhancing local inflammation and IEC damage. Aged A20 IEC/myel-KO mice (30-week and older) develop severe inflammation as evidenced by the thickening of the bowel wall ( Fig. 4a and Supplementary Fig. 2 ). On AB-PAS-stained A20 IEC/myel-KO colon sections, severe elongation of hyperproliferative Ki67+ crypts, lacking nearly all goblet cells, can be observed ( Fig. 4a,b ). CD45 immunostaining shows severe immune cell infiltration in colonic sections of A20 IEC/myel-KO mice ( Fig. 4c ). In line with previous observations in young A20 IEC/myel-KO mice ( Fig. 2e ), aged A20 IEC/myel-KO mice show pronounced epithelial apoptosis in colon tissue ( Fig. 4d ). Goblet cell loss, reduced mucin production and increased epithelial apoptosis severely affect the intestinal barrier, which compromises the spatial segregation of bacteria from the epithelial surface and even allows bacterial mucosal infiltration in A20 IEC/myel-KO mice ( Fig. 4e ). High-resolution endoscopy shows a granular and bleeding mucosal surface indicative of colitis in A20 IEC/myel-KO mice, in contrast to wild-type, A20 IEC-KO and A20 myel-KO mice, which display a healthy mucosal surface with normal vessel architecture ( Fig. 4f,g ). Finally, histological colitis scores, which were shown to be increased in young A20 IEC/myel-KO mice ( Fig. 1a ), increase to much higher levels in older (>30 weeks old) A20 IEC/myel-KO mice ( Fig. 4h ). 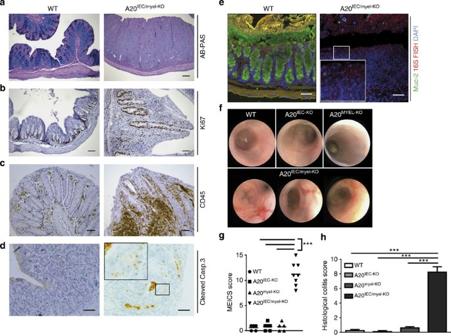Figure 4: Severe colitis in aged A20IEC/myel-KOmice. (a) representative images of AB-PAS stainings of colon sections from 30-week-old wild-type (WT) and A20IEC/myel-KOmice (Scale bars, 50 μm). (b–d) Immunostaining on colonic sections of wild-type (WT) and A20IEC/myel-KOmice for proliferating cells with Ki67 (b), infiltrating leukocytes with CD45 (c) and apoptotic cells with cleaved caspase-3 (d) antibodies (Scale bars,b: 50 μm,c: 20 μm,d: 50 μm). (e) Immunofluorescent staining for Muc-2 and 16S bacterial FISH on colonic sections from 30-week-old wild-type (WT) and A20IEC/myel-KOmice (Scale bars, 50 μm). (f) Representative endoscopic pictures of aged (>40 weeks) wild-type (WT), A20IEC-KO, A20myel-KOand A20IEC/myel-KOmice. (g) Colon inflammation detected by endoscopy is represented as MEICS score in aged (>40 weeks) wild-type (WT,n=5), A20IEC-KO(n=6), A20myel-KO(n=5) and A20IEC/myel-KO(n=8) mice. (h) Histological colitis scoring on aged wild-type (WT,n=8), A20IEC-KO(n=8), A20myel-KO(n=8) and A20IEC/myel-KO(n=8) mice showing strong colitis only in A20IEC/myel-KOmice. Error bars represent s.e.m. ***P<0.001 using Student’st-test. Figure 4: Severe colitis in aged A20 IEC/myel-KO mice. ( a ) representative images of AB-PAS stainings of colon sections from 30-week-old wild-type (WT) and A20 IEC/myel-KO mice (Scale bars, 50 μm). ( b – d ) Immunostaining on colonic sections of wild-type (WT) and A20 IEC/myel-KO mice for proliferating cells with Ki67 ( b ), infiltrating leukocytes with CD45 ( c ) and apoptotic cells with cleaved caspase-3 ( d ) antibodies (Scale bars, b : 50 μm, c : 20 μm, d : 50 μm). ( e ) Immunofluorescent staining for Muc-2 and 16S bacterial FISH on colonic sections from 30-week-old wild-type (WT) and A20 IEC/myel-KO mice (Scale bars, 50 μm). ( f ) Representative endoscopic pictures of aged (>40 weeks) wild-type (WT), A20 IEC-KO , A20 myel-KO and A20 IEC/myel-KO mice. ( g ) Colon inflammation detected by endoscopy is represented as MEICS score in aged (>40 weeks) wild-type (WT, n =5), A20 IEC-KO (n= 6), A20 myel-KO (n= 5) and A20 IEC/myel-KO (n= 8) mice. ( h ) Histological colitis scoring on aged wild-type (WT, n= 8), A20 IEC-KO (n= 8), A20 myel-KO (n= 8) and A20 IEC/myel-KO (n= 8) mice showing strong colitis only in A20 IEC/myel-KO mice. Error bars represent s.e.m. *** P <0.001 using Student’s t -test. Full size image Strikingly, A20 IEC/myel-KO mice older than 30 weeks of age often display tumour-like lesions in their colon (43%, n =44; Fig. 5a ). Indeed, endoscopic examination reveals multiple adenomatous polyps in old A20 IEC/myel-KO mice ( Fig. 5b ). Histological examination of affected regions shows a severely inflamed colonic mucosa containing dysplastic crypts, characterized by hyperproliferation, dysregulated crypt shape and orientation, loss of cell differentiation and low scale stratification ( Fig. 5c ). The tumours are however benign adenomas and do not invade submucosal tissue. Epithelial cells in these dysplastic tumour regions display elevated nuclear β-catenin and Sox9 expression ( Fig. 5d,e ), indicative for hyperactive Wnt signalling, and characteristic for colon adenoma development [17] . In addition, dysplastic crypt areas express Olfm4, which is a marker for murine small intestinal stem cells and is normally not observed in colon tissue of healthy mice, but is characteristic for human colon adenocarcinomas [18] ( Fig. 5f ). Together, we hypothesize that severe colitis and colorectal cancer development in aged A20 IEC/myel-KO mice is induced through continuous epithelial damage and regeneration, driven by cytotoxic factors released by hyperactive A20-deficient myeloid cells. We can however not exclude a contribution of other infiltrating immune cells, like T cells, to this phenotype. We therefore crossed A20 IEC/myel-KO mice into a Rag2-deficient background, generating mice also lacking functional T and B cells. A20 IEC/myel-KO Rag2 −/− mice, however, still display spontaneous IEC apoptosis both in small intestine and colon, similar to A20 IEC/myel-KO Rag2 +/− mice ( Fig. 6a ). A20 IEC/myel-KO Rag2 −/− mice also display small intestinal crypt hyperproliferation, as shown by Ki67 staining ( Fig. 6b ). In colon, A20 IEC/myel-KO Rag2 −/− mice already show clear signs of dysplasia, including misoriented star-shaped crypts, at an early age (15 weeks) compared with A20 IEC/myel-KO Rag2 +/− mice, which only display modest crypt hyperproliferation at this age ( Fig. 6b ). Leukocyte anti-CD45 staining does not show dramatic immune cell infiltration in ileal sections of 15-week-old A20 IEC/myel-KO Rag2 +/− and A20 IEC/myel-KO Rag2 −/− mice ( Fig. 6c , upper panel). In colon, however, immune cell staining is strongest in A20 IEC/myel-KO Rag2 −/− mice, where CD45+ cells surround dysplastic crypt areas ( Fig. 6c ). In conclusion, spontaneous intestinal defects observed in A20 IEC/myel-KO mice are preserved in Rag2-deficient conditions, indicating that functional T and B cells are dispensable for the inflammatory and tumorigenic phenotype of A20 IEC/myel-KO mice. Even more, A20 IEC/myel-KO Rag2 −/− mice develop much earlier severe colitis and dysplasia compared with A20 IEC/myel-KO Rag2 +/− littermates, suggesting rather protective activities of T and B cells in this context. Indeed, Rag2 −/− mice lack regulatory T cells (Tregs) and IgA-producing plasma cells which perform important immunoprotective functions in the intestine. 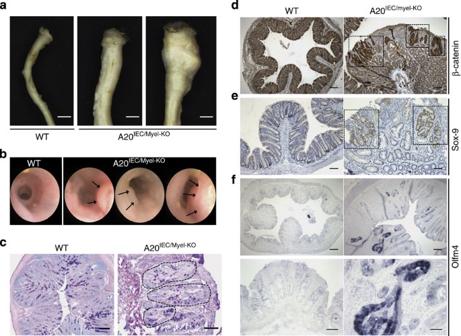Figure 5: Aged A20IEC/myel-KOmice develop colorectal tumours. (a) Representative macroscopic images of colons from 40-week-old wild-type (WT) and A20IEC/myel-KOmice (Scale bars, 5 mm). (b) Representative endoscopic images of 40-week-old wild-type (WT) and tumour-bearing A20IEC/myel-KOmice. Arrows indicate adenomatous neoplasms. (c) AB-PAS staining on colon sections of aged A20IEC/myel-KOmice. Dashed lines indicate dysplastic crypt areas (Scale bars, 100 μm left, 50 μm right). (d,e) Immunostaining on colon sections of aged wild-type (WT) and A20IEC/myel-KOmice for β-catenin (d) and Sox-9 (e) (Scale bars,d: 150 μm,e: 50 μm). Dashed squares indicate dysplastic areas with high β-catenin and Sox-9 expression. (f)In situhybridization for Olfm4 on colon sections from aged wild-type (WT) and A20IEC/myel-KOmice (Scale bars, upper 150 μm, lower 20 μm). Figure 5: Aged A20 IEC/myel-KO mice develop colorectal tumours. ( a ) Representative macroscopic images of colons from 40-week-old wild-type (WT) and A20 IEC/myel-KO mice (Scale bars, 5 mm). ( b ) Representative endoscopic images of 40-week-old wild-type (WT) and tumour-bearing A20 IEC/myel-KO mice. Arrows indicate adenomatous neoplasms. ( c ) AB-PAS staining on colon sections of aged A20 IEC/myel-KO mice. Dashed lines indicate dysplastic crypt areas (Scale bars, 100 μm left, 50 μm right). ( d , e ) Immunostaining on colon sections of aged wild-type (WT) and A20 IEC/myel-KO mice for β-catenin ( d ) and Sox-9 ( e ) (Scale bars, d : 150 μm, e : 50 μm). Dashed squares indicate dysplastic areas with high β-catenin and Sox-9 expression. ( f ) In situ hybridization for Olfm4 on colon sections from aged wild-type (WT) and A20 IEC/myel-KO mice (Scale bars, upper 150 μm, lower 20 μm). 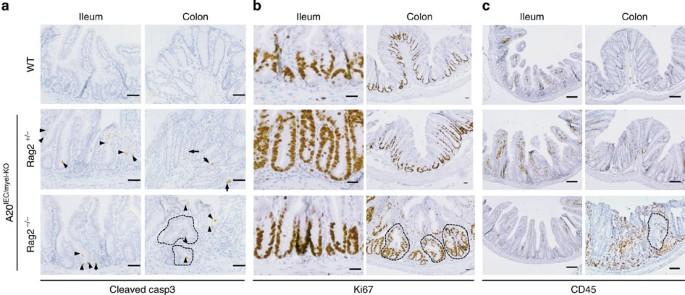Figure 6: Intestinal pathology is independent of B and T cells. (a–c) Representative images of ileal and colon sections of wild-type (WT), A20IEC/myel-KORag2+/−and A20IEC/myel-KORag2−/−mice immunostained for cleaved caspase-3 (a), Ki67 (b) and CD45 (c). Dashed lines indicate dysplastic crypt areas in colon (Scale bars,a: 50 μm,b: 25 μm,c: 50 μm). Full size image Figure 6: Intestinal pathology is independent of B and T cells. ( a – c ) Representative images of ileal and colon sections of wild-type (WT), A20 IEC/myel-KO Rag2 +/− and A20 IEC/myel-KO Rag2 −/− mice immunostained for cleaved caspase-3 ( a ), Ki67 ( b ) and CD45 ( c ). Dashed lines indicate dysplastic crypt areas in colon (Scale bars, a : 50 μm, b : 25 μm, c : 50 μm). Full size image A20 deficiency influences gut microbial composition Since the intestinal microbiome has profound effects on the immune system [19] and autoimmune pathologies including IBD are associated with changes in the composition of the intestinal microbiome [20] , we investigated to what extent bacterial communities were altered in the different A20 knockout mice. For this we performed 16S rDNA pyrosequencing analysis on caecal content from cohoused littermate wild-type, A20 IEC-KO , A20 myel-KO and A20 IEC/myel-KO mice. Enterocyte-specific A20 deficiency had no impact on intestinal microbial richness and composition ( Fig. 7 ), in accordance with the absence of any spontaneous phenotype in unchallenged A20 IEC-KO mice [8] . However, both A20 myel-KO and A20 IEC/myel-KO mice have significantly lower intestinal microbial richness compared with wild-type and A20 IEC-KO mice ( Fig. 7a , Supplementary Table 1 ). Although A20 myel-KO mice have no spontaneous intestinal phenotype, the observed dysbiosis may be linked to the rheumatoid arthritis-like phenotype of these mice [9] . Indeed, studies have shown that the inflammatory status of the host is inversely correlated to the richness of its microbial communities [21] , [22] . We observed that wild-type and A20 IEC-KO mice have more similar gut communities than A20 myel-KO and A20 IEC/myel-KO mice, suggesting the latter have less stable microbiotas due to their inflammatory phenotype ( Fig. 7b ). Nevertheless, A20 IEC/myel-KO microbiotas are still significantly different to those of A20 myel-KO mice in terms of composition ( Fig. 7b,c ; anosim P -value=0.048) and only A20 IEC/myel-KO mice are significantly different from the wild-type microbiota when taking into account bacterial phylogeny ( Supplementary Table 2 ). A20 IEC/myel-KO mice have increased abundance of Deferribacteres compared with the other three genotypes ( Fig. 7c ; P -value=0.009). Due to coprophagy, cage-effects can become non-negligible confounders in mice microbiota analysis [22] ( Supplementary Table 3 ). After controlling for gender-, age- and cage-effects, the Deferribacteres increase in A20 IEC/myel-KO mice is the only significant genotype-associated difference ( Fig. 7d , P -value=0.041 after multiple testing correction). This result is driven by a single-species assignment to Mucispirillum schaedleri , known to colonize the mucus layer of the gastrointestinal tract of rodents [23] . In this context, the Mucispirillum genus can be regarded as a biomarker for spontaneous colitis in A20 IEC/myel-KO mice. It remains currently unclear whether the observed dysbiosis solely develops in response to inflammation or actively contributes to the onset, maintenance and exacerbation of intestinal inflammation and neoplastic transformation in A20 IEC/myel-KO mice. 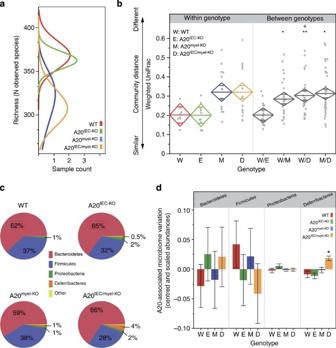Figure 7: A20 deficiency influences gut microbial composition. Microbiota analysis by 16S rDNA pyrosequencing of wild-type (WT), A20IEC-KO, A20myel-KOand A20IEC/myel-KOmice: (a) Distribution of observed microbiota richness. (b) Average weighted UniFrac distance (distance between communities on the basis of abundance and bacterial phylogenetics) within- and between-mouse genotypes. Anosim test with star phylogeny: *P<0.05, **P<0.001. Anosim with bacterial phylogenetic tree:+P<0.05. (c) Phylum-level comparisons of compiled samples. (d) Phylum-level abundance variation after controlling for cage-effects. Wilcoxon (BH correction). *P<0.05. W= WT, E=A20IEC-KO, M=A20myel-KOand D=A20IEC/myel-KO. Figure 7: A20 deficiency influences gut microbial composition. Microbiota analysis by 16S rDNA pyrosequencing of wild-type (WT), A20 IEC-KO , A20 myel-KO and A20 IEC/myel-KO mice: ( a ) Distribution of observed microbiota richness. ( b ) Average weighted UniFrac distance (distance between communities on the basis of abundance and bacterial phylogenetics) within- and between-mouse genotypes. Anosim test with star phylogeny: * P <0.05, ** P <0.001. Anosim with bacterial phylogenetic tree: + P <0.05. ( c ) Phylum-level comparisons of compiled samples. ( d ) Phylum-level abundance variation after controlling for cage-effects. Wilcoxon (BH correction). * P <0.05. W= WT, E=A20 IEC-KO , M=A20 myel-KO and D=A20 IEC/myel-KO . Full size image A20 polymorphisms and expression levels in human IBD patients Multiple SNPs in the A20 locus have previously been associated to inflammatory and autoimmune pathologies, including IBD [24] , [25] . To confirm the association of genetic variants in A20 to IBD, 17 of these SNPs were genotyped using Illumina custom chip in a cohort of 2,400 IBD patients (847 with UC and 1,553 with CD) and allele frequencies were compared with 921 healthy controls. None of these SNPs, however, showed genome-wide significance for association to IBD ( Supplementary Table 4 ). Strikingly, clear correlation between specific A20 polymorphisms and primary therapeutic response to anti-TNF (infliximab) therapy could be observed ( Table 1 ). Association for response to infliximab was seen with three intronic SNPs (rs6927210, rs 7753394, rs7773904), all in strong linkage disequilibrium ( r 2 =0.99). The strongest association was observed between carriers of the A allele of rs6927210 and response to infliximab ( P corr=0.036, odds ratio=1.335 (1.016–1.755)). This association remained significant (logistic regression analysis) after correction for disease (CD or UC) and disease location. Haplotype analysis revealed that the rs6927210 G–rs946227 G–rs7753394 A–rs7773904 C haplotype was associated with non-response to infliximab ( P =0.007, odds ratio=1.635 (1.140–2.345); Table 1 ). These data are in agreement with observations in psoriasis patients, where two SNPs in the A20 locus were associated to responsiveness to anti-TNF therapy [26] . Table 1 Polymorphisms associated with primary response to infliximab in IBD patients ( n =834). Full size table Since the SNPs associated to infliximab responsiveness are located in intronic sequences, they may affect regulatory elements which interfere with A20 expression. We therefore analyzed whether A20 expression in mucosal biopsies was linked to primary infliximab responsiveness, as previously described [27] . In colonic IBD, the mucosal expression of A20 was significantly lower in responders versus non-responders before treatment ( Supplementary Fig. 7 ). After infliximab therapy, expression was significantly downregulated in responders with complete mucosal healing, but not in non-responders. ( Supplementary Fig. 7 ). In contrast, no significant differences in A20 ileal expression were observed in CD patients with ileal disease ( Supplementary Fig. 7 ), but here sample size ( n =8) was lower than the sample size of the colonic IBD group ( n =20). Taken together, analysis of human patient samples identified A20 gene polymorphisms and mucosal expression levels as good prognostic markers for primary response to anti-TNF treatment. We hereby described a new mouse model of spontaneous intestinal inflammation and CAC, and shed light on the (patho)physiological importance of A20 in maintaining intestinal immune homeostasis. The functions of A20 are diverse and cell type-dependent: myeloid cells require A20 to prevent their spontaneous hyperactivation and expansion [9] , while IECs need A20 as a protective factor maintaining barrier stability in inflammatory conditions [8] . Although single IEC or myeloid deletion does not cause spontaneous intestinal defects, double IEC and myeloid A20 deficiency induces spontaneous intestinal pathology due to hyperinflammatory A20-deficient myeloid cells causing epithelial apoptosis and progressive loss of Paneth and goblet cells. Evidently, barrier destabilization caused by epithelial apoptosis combined with defective antimicrobial peptide and mucus production allows bacterial infiltration leading to more inflammation and damage to the epithelium ( Supplementary Fig. 8 ). This self-perpetuating condition causes severe inflammation and is strongest at sites with highest bacterial density, viz. in the colon, underscoring the involvement of infiltrating intestinal bacteria in the inflammatory pathology. These data thus identify A20 as the major anti-apoptotic protein indispensable for intestinal epithelial barrier stability and IEC survival during inflammation. Secretion of antimicrobial peptides by Paneth cells is an important protective mechanism by which intestinal immune homeostasis is established [28] , [29] , and defects in Paneth cell function have been described in IBD patients [30] , [31] and in multiple mouse lines, which develop spontaneous intestinal inflammation, such as Casp8 IEC-KO (ref. 32 ), FADD IEC-KO (ref. 33 ), NEMO IEC-KO (ref. 34 ) and IKK2ca IEC mice [35] . In addition, mice defective in ER stress signalling or autophagy, such as XBP1 IEC-KO mice [36] and hypomorphic ATG16L1 mice [37] , respectively, display Paneth cell abnormalities. Moreover, intestinal inflammation may even emerge from malfunctioning Paneth cells [38] . A20 deficiency in IECs does not cause spontaneous Paneth cell defects, but sensitizes their apoptotic loss in inflammatory conditions, either by direct low-dose TNF exposure or by exposure to cytokines produced by hyperactive A20-deficient myeloid cells, including TNF and IFNγ. Both these cytokines are well known for their cytotoxic activities on IECs and may contribute to the development of intestinal inflammation through their direct activity on Paneth cells [39] , [40] , [41] . Also goblet cells are severely affected in A20 IEC/myel-KO mice, compromising the protective epithelial mucus layer. Goblet cell depletion is also a frequent histopathological feature of IBD [42] , [43] , and goblet cells are also, due to their secretory character, highly sensitive to ER stress and inflammatory cytokines [36] . The early loss of Paneth and goblet cells in A20 IEC/myel-KO mice and subsequent reduction in innate defence may thus sensitize these mice to the development of intestinal inflammation. CAC is the most serious complication of IBD, and it is now well accepted that chronic inflammation drives neoplastic transformation of the intestinal epithelium [2] , [44] . NF-κB activation in IECs may promote CAC development by driving the expression of pro-survival genes, and growth factors creating a tumour-promoting microenvironment [35] , [45] , [46] . Moreover, NF-κB can enhance Wnt activation and induce dedifferentiation of non-stem cells that acquire tumour-initiating capacity [47] , therefore chronic NF-κB activation can bypass the requirement of Wnt activating mutations during early CAC development. In addition, ROS production and NF-κB signalling facilitate Wnt-driven stem-cell proliferation and transformation initiating colon cancer development [48] . A20 IEC/myel-KO mice develop colorectal adenomas with dysplastic regions characterized by increased expression of β-catenin and Sox9, indicative of a hyperactive Wnt signalling, and by the expression of the intestinal stem cell marker Olfm4, which is characteristic for a subset of human colorectal cancers [18] . A recent study reported a role for A20 in restricting Wnt signalling suppressing colorectal cancer development [16] . Our data, however, do not suggest a direct role for A20 in Wnt inhibition, since we did not observe enhanced Wnt activation in IECs from A20 IEC-KO mice or in tumour-free areas from A20 IEC/myel-KO mice. We therefore believe that aberrant Wnt activation in dysplastic crypt foci is caused by secondary events due to chronic inflammation. Finally, T and B cells are dispensable for the development of intestinal inflammation and dysplasia in A20 IEC/myel-KO mice. A20 IEC/myel-KO Rag2 −/− mice develop an even more severe and earlier intestinal inflammation and dysplasia compared with A20 IEC/myel-KO mice, indicating protective functions for the adaptive immune system in this model. In this respect, A20 IEC/myel-KO Rag2 −/− mice resemble TRUC (Tbet- and Rag2-deficient UC) mice, which develop severe colitis and CAC induced by hyperactive dendritic cells and innate lymphoid cells in the absence of protective T and B cell responses [49] , [50] , [51] . To translate the above described findings to humans, samples from a large cohort of IBD patients were analyzed. Indeed, A20 polymorphisms have been associated to multiple inflammatory pathologies including IBD [24] , [25] . Although none of the published A20 SNPs showed genome-wide significance for susceptibility to IBD, we found specific haplotypes to be associated with non-response to infliximab. In addition, lower expression levels of A20 seem predictive of primary response to infliximab, while non-responders display significantly higher and stable A20 expression levels. These data are in line with studies in rheumatoid arthritis patients [52] and Crohn’s disease patients [53] where low A20 expression has been correlated to good anti-TNF response. Taken together, we identified A20 as a potential biomarker for the prognosis of anti-TNF therapy. Since 10–20% of IBD patients fail to respond to initial anti-TNF treatment, early identification of non-responsive patients is of great medical and socioeconomic value. Generation of tissue-specific A20-deficient mice Conditional A20/ tnfaip3 knockout mice, in which exons IV and V of tnfaip3 gene are flanked by two LoxP sites, were previously described [8] . A20 floxed (A20 FL/FL ) mice were crossed with LysM-Cre transgenic mice [54] generating myeloid-specific A20 knockout mice (A20 myel-KO , A20 FL/FL LysMCre Tg/+ ), or with Villin-Cre transgenic mice [55] generating IEC-specific A20 knockout mice (A20 IEC-KO , A20 FL/FL VillinCre Tg/+ ). A20 myel-KO and A20 IEC-KO mice were intercrossed generating mice lacking A20 both in myeloid cells and IECs (A20 IEC/myel-KO , A20 FL/FL VillinCre Tg/+ LysMCre Tg/+ ). As wild-type (WT) controls, A20 floxed (A20 FL/FL VillinCre +/+ LysMCre +/+ ) sex-matched littermate mice were used in all studies. Experiments were performed on both male and female mice backcrossed into the C57BL/6 genetic background for at least four generations. Mice were housed in individually ventilated cages in a specific pathogen-free facility. All experiments on mice were conducted according to institutional, national and European animal regulations. Animal protocols were approved by the ethics committee of Ghent University. Histological colitis score Histopathology was scored as described earlier [56] . Briefly, colitis scores were determined as averages of six histological parameters (goblet cell loss, crypt abscesses, mucosal hyperaemia, cellular infiltration in the lamina propria, mucosal elongation and epithelial erosion), with scores according to a scale as follows: 0, normal histology; 1, mild pathology for each histological parameter; 2, moderate pathology; and 3, severe pathology. Histological scores of the proximal, middle and distal portion of the colons were determined, and the average was calculated. Stool colitis score A20 myel-KO , A20 IEC-KO , A20 IEC/myel-KO and littermate wild-type controls were scored for stool consistency and faecal blood loss using Hemoccult-Sensa (Beckman Coulter Inc.). For bleeding, a score of 0 was assigned for no blood, 2 for positive hemoccult and 4 for gross bleeding. For stool consistency, a score of 0 was assigned for well-formed pellets; pasty and semiformed stools were scored as 2 and liquid stools as 4. These scores were added together and divided by 2, resulting in a clinical score ranging from 0 (healthy) to 4 (maximal colitis). To eliminate any diagnostic bias, mice were scored blindly. Endoscopic analysis High-resolution mouse endoscopy and murine endoscopic index of colitis severity (MEICS) scoring was performed, as previously described [57] , using a ‘Coloview’ endoscopic system (Karl Storz, Tuttlingen, Germany). Mice were anaesthetized with 2–2.5% isoflurane in oxygen during endoscopy. Isolation of intestinal crypts and three-dimensional organoid culture Intestinal organoids were derived from small intestine as previously described [58] . Briefly, a 5 cm piece of duodenum/jejunum was dissected and washed in phosphate-buffered saline (PBS). The intestine was opened longitudinally, villi were scraped away and the tissue was chopped in 2–3 mm pieces. After thorough washing in PBS, pieces were incubated in 2 mM EDTA/PBS for 30 min at 4 °C on a rocking platform. After passage through a 70-μm cell strainer, crypt fractions were isolated and purified by successive centrifugation steps. One ml of matrigel (BD Biosciences) was added to a pellet of 100–1,000 crypts, and drops of 50 μl crypt-containing matrigel were added to pre-warmed wells in a 24-well plate. After polymerization, 500 μl complete growth medium containing EGF (Peprotech), R-Spondin1 (R&D) and Noggin (Peprotech) [59] was added to each well every 2 days. For Wnt3a stimulation, growth medium was replaced with R-spondin-free medium 8 h before stimulation. A total of 200 ng ml −1 Wnt3a (Peprotech) was added in R-spondin containing growth medium for stimulation. For TNF and IFNγ stimulation ( Escherichia coli -derived recombinant protein produced by VIB-Protein service facility), 10 ng ml −1 TNF or IFNγ was diluted in organoid growth medium. Quantification of cytokines Cytokines in serum were quantified by the Bio-plex Pro kit (Bio-Rad) on the Bio-plex 200 system (Bio-rad). Flow cytometry Flow cytometric analysis was performed on a LSRII (BD Biosciences). Cell suspensions were prepared from total spleens. Red blood cells were lysed by incubation with ACK lysis buffer (BioWhittaker). Total cell suspensions were pre-incubated with purified rat anti-mouse CD16/CD32 (mouse Fc block; BD Biosciences, Pharmingen, 2.5 μg ml −1 ), and splenocytes were incubated with anti-CD11b-PerCpCy5.5 and anti-Gr1-FITC (BD Biosciences, both 1 μg ml −1 ). Tissue sample preparation Freshly isolated colonic and ileal segments were flushed with PBS to remove the faecal content and subsequently flushed with formalin (4% formaldehyde in PBS and fixed by overnight incubation in a 10-fold excess of formalin at 4 °C. Formalin was removed and intestines were washed twice with PBS before embedding in paraffin wax using standard methods. Histology Formalin fixed tissue was embedded in paraffin and 4 μm tissue sections were cut and stained with haematoxylin/eosin. For combined AB and PAS stainings, dewaxed sections were hydrated and incubated in AB for 20 min. Sections were subsequently washed with water before incubation in 1% periodic acid for 10 min followed by incubation in Schiff’s reagent for 10 min. Sections were counterstained with Mayer’s haematoxylin for 30 s, washed and dehydrated before mounting with Pertex. For immunochemistry, sections were dewaxed and incubated in Dako antigen retrieval solution and boiled for 20 min in a Pick cell cooking unit and cooled down for 2.5 h. Endogenous peroxidase activity was blocked by immersing slides in peroxidase-blocking buffer (0.040 M citric acid, 0.121 M disodium hydrogen phosphate, 0.030 M sodium azide, 1.5% hydrogen peroxide) for 15 min at room temperature. Blocking buffer (1% bovine serum albumin in PBS) was added to the slides for 30 min at room temperature. Primary antibodies (mouse anti-β-catenin, 1/50 dilution, Transduction Lab; rabbit anti-Sox-9, 1/600 dilution, Chemicon; mouse anti-Ki67, 1/100 dilution, Novocastra; rabbit anti-lysozyme, 1/1,000 dilution, Dako; anti-Cleaved caspase-3, 1/1,000 dilution, Cell Signaling; anti-CD45, 1/1,000 dilution, BD Pharmingen) were incubated overnight in bovine serum albumin in PBS. Slides were then incubated with secondary antibody (polymer horseradish peroxidase-labelled anti-mouse/rabbit, Envision) and peroxidase was detected by diaminobutyric acid (DAB) substrate. Slides were counterstained with Mayer's haematoxylin and mounted in Pertex mounting medium. For lysozyme staining, sections were incubated with DyLight-488 conjugated goat anti-rabbit secondary antibodies (1:1,000 dilution, Fisher Bioblock Scientific), and cell nuclei were counterstained with DAPI (4′,6-diamidino-2-phenylindole, Invitrogen) in ProLong Gold anti-fade reagent. Apoptosis was analyzed with an in situ cell death detection kit (TMR-red, Roche) after antigen retrieval before incubation with the primary anti-lysozyme antibody for combined TUNEL-lysozyme-DAPI staining. Fluorescence Microscopy was performed using a TCS SP5 confocal microscope (Leica). Confocal images were represented as frontal views of three-dimensional images (3D Opacity) or as three-dimensional projections (Extended focus), using Volocity 5.5 imaging software (PerkinElmer). Quantification of cleaved caspase-3 positive cells Ileal and colonic sections at four different positions were analyzed per mouse, 10 consecutive crypts within each section were analyzed for presence of cleaved caspase-3 positive cells and averages per crypt are displayed. In situ hybridization The 4 μm-thick sections were rehydrated as described and treated with 0.2 M sodium chloride and proteinase K. Slides were post-fixed, and sections were demethylated with acetic anhydride and prehybridized. Hybridization was carried out in a humid chamber with 500 ng ml −1 of freshly prepared digoxigenin-labelled Olfm4 RNA probe (image clone 1078130) or Cryptidin-1 RNA probe (image clone 1096215) for at least 48 h at 68 °C. Slides were then washed and incubated with secondary anti-digoxigenin antibody (Roche) at 4 °C overnight, and developed using nitro blue tetrazolium chloride/5-bromo-4-chloro-3-indolyl-phosphate. Mucin immunostaining and bacterial FISH Stainings were performed as described [10] . Briefly, tissue was fixed in methanol-Carnoy (60% dry methanol, 30% chloroform, 10% glacial acetic acid) solution overnight, and 4 μm paraffin sections were processed for Mucin-2 immunohistochemistry (Santa Cruz, sc-15334, 1:200 dilution) and bacteria were detected with the universal bacterial FISH probe EUB338 (5′- GCTGCCTCCCGTAGGAGT -3′), with 5′Cy3 labelling. Quantitative real-time PCR Ileal segments of 5 cm long were freshly isolated and flushed with PBS to remove the faecal content. One end was ligated and filled with RNA lysis buffer (Aurum Total RNA Mini kit, Bio-Rad Laboratories) on ice for 5 min. RNA was purified using the Aurum Total RNA Mini kit (Bio-Rad Laboratories) and cDNA synthesis was performed using the iScript cDNA synthesis kit (Bio-Rad Laboratories) according to the manufacturer’s instructions. Ten nanograms of cDNA was used for quantitative PCR in a total volume of 10 μl with LightCycler 480 SYBR Green I Master Mix (Roche) on a LightCycler 480 (Roche). Real-time PCR reactions were performed in triplicates. The following mouse-specific primers were used: ubiquitin forward, 5′- AGGTCAAACAGGAAGACAGACGTA -3′; ubiquitin reverse, 5′- TCACACCCAAGAACAAGCACA -3′; lysozyme-P forward, 5′- gccaaggtctaacaatcgttgtgagttg -3′; lysozyme-P reverse, 5′- cagtcagccagcttgacaccacg -3′; cryptidin-1 forward, 5′- tcaagaggctgcaaaggaagagaac -3′; cryptidin-1 reverse, 5′- tggtctccatgttcagcgacagc -3′. Ascl-2 forward 5′- CATGGAAGCACACCTTGACTG -3′; Ascl-2 reverse 5′- CATCAAGCTTGCATTCAGCC -3′; CD44 forward 5′- TCTGCCATCTAGCACTAAGAGC -3′; CD44 reverse 5′- GTCTGGGTATTGAAAGGTGTAGC -3′; TnfRsF19 forward 5′- ATTCTCTTCCTACTCCACCTG -3′; TnfRsF19 5′- CATAGCCGAAGCCACATTC -3′; Lgr5 forward 5′- AGAACACTGACTTTGAATGG -3′; Lgr5 reverse 5′- GACAAATCTAGCACTTGGAG -3′; Olfm4 forward 5′- CGAAGTGGAGATAAGGAATATGAC -3′; Olfm4 reverse 5′- CCTCACATTCTTTCAGCTTGG -3′. Electron microscopy. Intestinal tissue was washed twice for 30 min in sodium cacodylate buffer (0.1 M pH 7.3, Sigma Genosys) embedded in agarose (Sigma Genosys type VII, catalogue no. A-4018), and sectioned at 500 μm and placed in PBS. Tissue was dissected out and osmicated for 1 h at room temperature in 2% OsO 4 in sodium cacodylate buffer. Samples were dehydrated through a graded ethanol series, followed by embedding in Spurr’s resin. Ultrathin sections of a gold interference colour were cut using an ultramicrotome (Leica EM UC6), followed by poststaining with uranyl acetate for 40 min and for 7 min in lead citrate in a Leica EM AC20 and collected on formvar-coated copper slot grids. They were viewed with a transmission electron microscope JEOL 1010 (JEOL, Tokyo, Japan). In vivo TNF treatment Mice were injected intraperitoneally with a sublethal dose of mouse TNF (1 μg TNF per 20 g body weight). E. coli -derived recombinant mTNF had a specific activity of 9.46 × 10E7 IU mg −1 . Mouse TNF was produced and purified to homogeneity in our laboratory, and endotoxin levels did not exceed 1 ng mg −1 of protein. Mice were euthanized after 4 h for histological analysis. TNFAIP3 SNP and expression analysis in human IBD samples TNFAIP3 genetic variants were evaluated in 2400 IBD patients from the IBD unit of the University Hospital of Leuven (847 with UC and 1,553 with CD) and compared with allele frequencies of 921 non-IBD controls. Both patients and controls were genotyped through the immunochip platform. Allele frequencies were calculated with the software package PLINK [60] and the Cochran-Armitage trend test was used to compare frequencies. Logistic regression analysis was performed to correct associations for disease (UC or CD) and disease location (ileal, colonic or ileocolonic). Genome-wide significance was determined as P =5 × 10 −8 . Haplotype analysis was performed with the software package Haploview [61] . Primary non-response in those patients that received infliximab was assessed by experienced clinicians and defined as no improvement of clinical symptoms after 2 or 3 infusions. A20 expression was investigated in endoscopically-derived intestinal mucosal biopsies, as described by Arijs et al . [27] , from 61 active IBD patients naive to infliximab therapy before and 4 to 6 weeks after their first infliximab infusion and from 12 normal controls. Response was defined on the basis of endoscopic and histologic findings. TNFAIP3 gene expression was analyzed by two probe sets (202643_s_at and 202644_s_at) on the array. Microbiota analysis Total DNA was extracted from mice caecal content using the QIAamp DNA stool Mini kit (Qiagen). DNA samples were amplified by 454/Roche Titanium pyrosequencing of the V3–V5 16S RDNA region (BGI, Shenzhen). The Qiime pipeline [62] was used for open-reference OTU picking with (USEARCH v7) [63] , obtaining a sample-wise OTU abundance matrix (630 OTU, 22 samples) with Greengenes [64] (version 13_5) taxonomic assignment. Statistical analyses were performed in R (package phyloseq [65] ). Variation partitioning and partialling out of gender, age and cage-effects were performed by redundancy analysis (RDA). Statistics Results are expressed as the mean±s.e.m. Statistical significance between experimental groups was assessed using the Wilcoxon signed-rank test for paired samples and the using Student’s t -test or Mann–Whitney U -test for unpaired samples. How to cite this article: Vereecke, L. et al . A20 controls intestinal homeostasis through cell-specific activities. Nat. Commun. 5:5103 doi: 10.1038/ncomms6103 (2014).